A spatial emergent constraint on the sensitivity of soil carbon turnover to global warming Carbon cycle feedbacks represent large uncertainties in climate change projections, and the response of soil carbon to climate change contributes the greatest uncertainty to this. Future changes in soil carbon depend on changes in litter and root inputs from plants and especially on reductions in the turnover time of soil carbon ( τ s ) with warming. An approximation to the latter term for the top one metre of soil (Δ C s,τ ) can be diagnosed from projections made with the CMIP6 and CMIP5 Earth System Models (ESMs), and is found to span a large range even at 2 °C of global warming (−196 ± 117 PgC). Here, we present a constraint on Δ C s,τ , which makes use of current heterotrophic respiration and the spatial variability of τ s inferred from observations. This spatial emergent constraint allows us to halve the uncertainty in Δ C s,τ at 2 °C to −232 ± 52 PgC. Climate–carbon cycle feedbacks [1] must be understood and quantified if the Paris Agreement Targets are to be met [2] . Changes in soil carbon represent a particularly large uncertainty [3] , [4] , [5] , [6] , [7] , with the potential to significantly reduce the carbon budget for climate stabilisation at 2 °C global warming [8] . Previous studies have investigated the response of soil carbon to climate change based on both observational studies [9] and Earth System Models (ESMs) [10] . ESMs are coupled models which simulate both climate and carbon cycle processes. Projects such as the Coupled Model Inter-comparison Project (CMIP) [11] , [12] , have allowed for consistent comparison of the response of soil carbon under climate change from existing state-of-the-art ESMs. However, the uncertainty due to the soil carbon feedback did not reduce significantly between the CMIP3 and CMIP5 model generations [6] , or with the latest CMIP6 models (see Fig. 1 and Supplementary Fig. 1 ), such that the projected change in global soil carbon still varies significantly amongst models [13] . Fig. 1: Uncertainty in future changes in soil carbon due to reduction in turnover time. Δ C s,τ vs. Δ T plot diagnosed from sixteen Earth System Models (seven CMIP6 ESMs and nine CMIP5 ESMs), for three different future scenarios: SSP126, SSP245, SSP585, or RCP2.6, RCP4.5, RCP8.5, respectively. a The change in soil carbon due to the change in soil carbon turnover time against change in global mean temperatures; b The fractional change in soil carbon due to the change in soil carbon turnover time against change in global mean temperatures, and compared to different effective q 10 sensitivities. Full size image This study uses an alternative method to obtain a constraint on the ESM projections of soil carbon change. In previous studies, emergent constraints based on temporal trends and variations have been used successfully to reduce uncertainty in climate change projections [14] . Our approach follows the method used in Chadburn et al. [15] , where a spatial temperature sensitivity is used to constrain the future response to climate change—which we term as a spatial emergent constraint . Our study combines the Chadburn et al. [15] method with the soil carbon turnover analysis of Koven et al. [16] to get a constraint on the sensitivity of soil carbon turnover to global warming. Soil carbon ( C s ) is increased by the flux of organic carbon into the soil from plant litter and roots, and decreased by the breakdown of that organic matter by soil microbes which releases CO 2 to the atmosphere as the heterotrophic respiration flux ( R h ). If the vegetation carbon is at steady-state, litter-fall will equal the Net Primary Production of plants (NPP). If the soil carbon is also near to a steady-state—and in the absence of significant fire fluxes and other non-respiratory carbon losses—the litter-fall, NPP, and R h will be approximately equal to one another. Even over the historical period, when atmospheric CO 2 has been increasing and there has been a net land carbon sink, this approximation holds well (see Supplementary Fig. 4 ). In order to separate the effects of changes in NPP from the effects of climate change on R h , we define an effective turnover time [17] for soil carbon as τ s = C s / R h . The turnover time of soil carbon is known to be especially dependent on temperature [3] . A common assumption is that τ s decreases by about 7% per °C of warming (equivalent to assuming that q 10 = 2) [18] . However, this sensitivity differs between models, and also between models and observations. We can write a long-term change in soil carbon (Δ C s ), as the sum of a term arising from changes in litter-fall (Δ C s,L ), and a term arising from changes in the turnover time of soil carbon (Δ C s,τ ): 
    ΔC_s= Δ(R_h τ_s)≈ΔC_s,L(t)+ΔC_s,τ(t) = τ_s,0 ΔR_h(t)+R_h,0 Δτ_s(t)
 (1) Model projections of the first term (Δ C s,L ) differ primarily because of differences in the extent of CO 2 -fertilisation of NPP, and associated nutrient limitations. The second term (Δ C s,τ ) differs across models because of differences in the predicted future warming, and because of differences in the sensitivity of soil carbon decomposition to temperature (which includes an influence from faster equilibration of fast-turnover compared to slow-turnover carbon pools under changing inputs [13] ). This study provides an observational constraint on the latter uncertainty. As the vast majority of the CMIP6 and CMIP5 models do not yet represent vertically resolved deep soil carbon in permafrost or peatlands, we focus our constraint on carbon change in the top 1 metre of soil. To ensure a fair like-for-like comparison we also exclude the two CMIP6 models that do represent vertically-resolved soil carbon (CESM2 and NorESM2), although this has a negligible effect on our overall result. Our study therefore applies to soil carbon loss in the top 1 metre of soil only. Below we show that it is possible to significantly reduce the uncertainty in this key feedback to climate change using current-day spatial data to constrain the sensitivity to future warming. Proof of concept For each ESM, we begin by calculating the effective τ s using time-averaged (1995–2005) values of C s and R h at each grid-point, and applying our definition of τ s = C s / R h . We do likewise for observational datasets of soil carbon in the top 1 metre [19] , [20] and time-averaged (2001–2010) heterotrophic respiration [21] , as shown in Fig. 2 . Figure 2 c shows the map of inferred values of τ s from these observations, with a notable increase from approximately 7 years in the warm tropics to over 100 years in the cooler high northern latitudes. 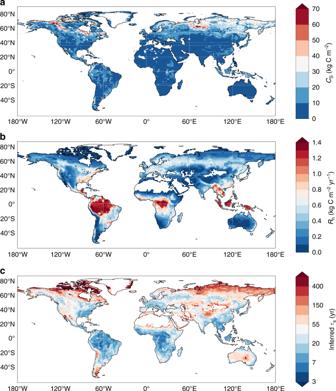Fig. 2: Spatial variability of soil carbon turnover time inferred from observations. Maps ofaobserved soil carbon (Cs) to a depth of 1 m (kg C m−2)19,20,bobserved heterotrophic respiration (Rh,0) (kg C m−2yr−1)21, andcinferred soil carbon turnover time (\(\mathrm{log}\,{\tau }_{{\rm{s}}}\)) (yr). Fig. 2: Spatial variability of soil carbon turnover time inferred from observations. Maps of a observed soil carbon ( C s ) to a depth of 1 m (kg C m −2 ) [19] , [20] , b observed heterotrophic respiration ( R h,0 ) (kg C m −2 yr −1 ) [21] , and c inferred soil carbon turnover time ( \(\mathrm{log}\,{\tau }_{{\rm{s}}}\) ) (yr). Full size image Similar maps can be diagnosed for each of year of data, for each ESM, and for each future scenario, giving time and space varying values of τ s for each model run. This allows us to estimate Δ C s,τ , via the last term on the right of Eq. ( 1 ). For each ESM, the R h,0 value is taken as the mean over the decade 1995–2005, to overlap with the time period of the observations and to maintain consistency across CMIP generations. Individual grid-point τ s values are calculated for each year before calculating area-weighted global totals of Δ C s,τ . The uncertainty of Δ C s,τ stems from the uncertainty in soil carbon turnover ( τ s ), and the uncertainty due to differing climate sensitivities of the models. In this study, we aim to quantify and constrain the uncertainty in τ s . To isolate the latter uncertainty, we consider Δ C s,τ for differing levels of global mean warming in each model. The resulting dependence of global total Δ C s,τ on global warming is shown in Fig. 1 a, for each of the ESMs considered in both CMIP6 and CMIP5 (seven CMIP6 ESMs and nine CMIP5 ESMs), and for three Shared Socioeconomic Pathways (SSP): SSP126, SSP245 and SSP585 (CMIP6) [22] , or the equivalent Representative Concentration Pathways (RCP): RCP2.6, RCP4.5 and RCP8.5 (CMIP5) [23] . In all cases Δ C s,τ is negative, which is consistent with the soil carbon turnover time decreasing with warming. 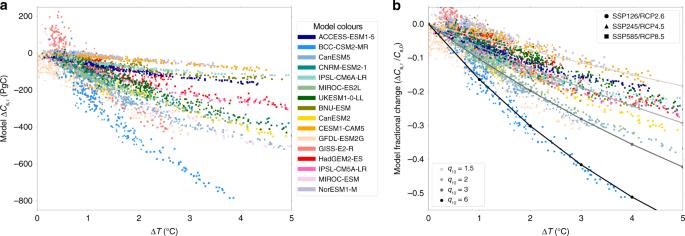The more surprising thing to note is the huge range in the projections, with a spread at 2 °C global mean warming of approximately 400 PgC, regardless of future SSP/RCP scenario. Fig. 1: Uncertainty in future changes in soil carbon due to reduction in turnover time. ΔCs,τvs. ΔTplot diagnosed from sixteen Earth System Models (seven CMIP6 ESMs and nine CMIP5 ESMs), for three different future scenarios: SSP126, SSP245, SSP585, or RCP2.6, RCP4.5, RCP8.5, respectively.aThe change in soil carbon due to the change in soil carbon turnover time against change in global mean temperatures;bThe fractional change in soil carbon due to the change in soil carbon turnover time against change in global mean temperatures, and compared to different effective q10sensitivities. Figure 1 b plots the fractional change in soil carbon Δ C s,τ / C s,0 , showing that there is a large range of effective q 10 sensitivities between the model projections. Unfortunately, we do not have time-varying observational datasets of C s and R h that might allow us to directly constrain this projection uncertainty. Instead we explore whether the observed spatial variability in τ s (as shown in Fig. 2 c) provides some observational constraint on the sensitivity of τ s to temperature. In doing so, we are motivated by Chadburn et al. [15] who used the correlation between the observed geographical distributions of permafrost and air temperature to constrain projections of future permafrost area under global warming. Similarly, we use ESMs to test whether the spatial variation in τ s reveals the sensitivity of soil carbon turnover to temperature. The spatial patterns of τ s in CMIP5 simulations and observations were previously shown in Koven et al. [16] , and here we test whether such relationships can be used to estimate the response of soil carbon to future climate change, using a combination of CMIP6 and CMIP5 models. 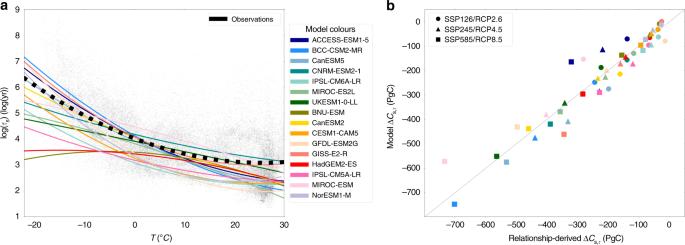Fig. 3: Using spatial variability of soil carbon turnover time to estimate ΔCs,τ. aScatter-plot of the relationship between\(\mathrm{log}\,{\tau }_{{\rm{s}}}\)and mean air temperature from observations19,20,21,24(black points), and a quadratic fit (black-dotted line) representing the observational temperature sensitivity of\(\mathrm{log}\,{\tau }_{{\rm{s}}}\). The equivalent quadratic fits for the ESMs are shown by the coloured lines;bThe proof of principle for our method, showing an actual vs. estimated comparison, representing the modelled versus the relationship-derived values of the ΔCs,τ, where the change is considered between the start (1995–2005) and the end (2090–2100) of 21st century and is assumed to relate to the top 1 metre of soil. Figure 3 a is a scatter plot of \(\mathrm{log}\,{\tau }_{{\rm{s}}}\) against temperature, using the τ s values shown in Fig. 2 c and mean temperatures from the WFDEI dataset over the period 2001–2010 [24] . The thick black-dotted line is a quadratic fit through these points. Also shown for comparison are equivalent quadratic fits for each model (coloured lines), using the model \(\mathrm{log}\,{\tau }_{{\rm{s}}}\) and mean near-surface air temperature ( T ) values for each grid-point, over an overlapping period with the observations (1995–2005). There is a spread in the individual data points due to variation in soil moisture, soil type, and other soil parameters [25] . The model specific spread in the data can be seen for the CMIP6 and CMIP5 models in Supplementary Figs. 2 and 3 , respectively. Although models do not account for every possible factor contributing to this spread, the spread of points in the models is generally similar to the observations. However, differences between the best-fit functions relating τ s to T are evident between the models, and between the models and the observations [16] . Fig. 3: Using spatial variability of soil carbon turnover time to estimate Δ C s,τ . a Scatter-plot of the relationship between \(\mathrm{log}\,{\tau }_{{\rm{s}}}\) and mean air temperature from observations [19] , [20] , [21] , [24] (black points), and a quadratic fit (black-dotted line) representing the observational temperature sensitivity of \(\mathrm{log}\,{\tau }_{{\rm{s}}}\) . The equivalent quadratic fits for the ESMs are shown by the coloured lines; b The proof of principle for our method, showing an actual vs. estimated comparison, representing the modelled versus the relationship-derived values of the Δ C s,τ , where the change is considered between the start (1995–2005) and the end (2090–2100) of 21st century and is assumed to relate to the top 1 metre of soil. Full size image This suggests that we may be able to constrain Δ C s,τ using the observed τ s vs. T fit from the observations, but only if we can show that such functions can be used to predict Δ C s,τ under climate change. In order to test that premise, we attempt to reconstruct the time-varying Δ C s,τ projection for each model using the time-invariant τ s vs. T fit across spatial points (Fig. 3 a), and the time-invariant R h,0 field. The change in soil carbon turnover time (Δ τ s (t)) for a given model run is estimated at each point based-on the τ s vs. T curve, and the time-varying projection of T at that point. A local estimate of the subsequent change in soil carbon can then be made based-on the farthest right-hand term of Eq. ( 1 ) ( R h,0 Δ τ s ), which can be integrated up to provide an estimated change in global soil carbon in the top 1 metre (Δ C s,τ ). Figure 3 b shows the result of this test for all models and all respective SSP/RCP scenarios. The axes of this plot show equivalent variables which represent the global Δ C s,τ between the mean value for 2090–2100 and the mean value for 1995–2005. The y -axis represents the actual values for each model as shown in Fig. 1 , and the x -axis represents our estimate derived from spatial variability (as in Fig. 3 a). As hoped, actual vs. estimated values cluster tightly around a one-to-one line with an r 2 correlation coefficient value of 0.90. Although some hot-climate regions will inevitably experience temperatures beyond those covered by current-day spatial variability, these tend to be regions with low soil carbon, so this does not have a major impact on the success of our method. Spatial emergent constraint This gives us confidence to use the τ s vs. T fit and R h,0 from observations to constrain future projections of Δ C s,τ . To remove the uncertainty in future Δ C s,τ due to the climate sensitivity of the models, we investigate a common amount of global mean warming in each model. 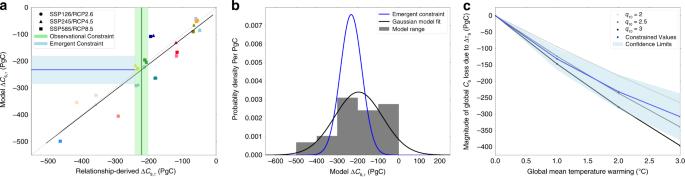Fig. 4: Emergent constraint on ΔCs,τas a function of global warming. aActual vs. estimated scatter plot for ΔCs,τfor 2 °C of global warming. The vertical green line defines the observational constraint which is derived using observational data and the future spatial temperature field of each model (decadal average), and the shaded region represents the corresponding uncertainty (±1 standard deviation). The horizontal blue line represents our emergent constraint, with the shaded region showing the corresponding uncertainty (±1 standard deviation) which results from the differing future spatial warming patterns seen in the future spatial temperature fields across the ESMs, and the emergent relationship between the model data points (black line).bProbability density function showing the Gaussian distribution of ΔCs,τvalues from the unweighted prior model ensemble (black line) and the emergent constraint (blue line).cConstrained ΔCs,τvalues at different levels of global warming (blue), including the likely (±1 standard deviation) uncertainty bounds (shaded blue). Different effective global q10values shown for comparison; our emergent constraint is consistent with an effective q10≈ 2.5 ± 0.6. Figure 4 a is similar to Fig. 3 b but instead for the more policy-relevant case of 2 °C of global warming. As before, the y -axis represents the modelled Δ C s,τ , and the x -axis is our estimate derived from spatial variability. Once again, the actual and estimated values of Δ C s,τ cluster around the one-to-one line (with r 2 = 0.87). The model range arises partly from differences in the initial field of heterotrophic respiration ( R h,0 ), and partly from differences in Δ τ s (compare first row to penultimate row of Table 1 ). Fig. 4: Emergent constraint on Δ C s,τ as a function of global warming. a Actual vs. estimated scatter plot for Δ C s,τ for 2 °C of global warming. The vertical green line defines the observational constraint which is derived using observational data and the future spatial temperature field of each model (decadal average), and the shaded region represents the corresponding uncertainty (±1 standard deviation). The horizontal blue line represents our emergent constraint, with the shaded region showing the corresponding uncertainty (±1 standard deviation) which results from the differing future spatial warming patterns seen in the future spatial temperature fields across the ESMs, and the emergent relationship between the model data points (black line). b Probability density function showing the Gaussian distribution of Δ C s,τ values from the unweighted prior model ensemble (black line) and the emergent constraint (blue line). c Constrained Δ C s,τ values at different levels of global warming (blue), including the likely (±1 standard deviation) uncertainty bounds (shaded blue). Different effective global q 10 values shown for comparison; our emergent constraint is consistent with an effective q 10 ≈ 2.5 ± 0.6. Full size image Table 1 Sensitivity study of spatial emergent constraint. Full size table The vertical green line in Fig. 4 a represents the mean estimate when the τ s vs. T relationship and the R h,0 field from the model are replaced with the equivalents from the observations. The spread shown by the shaded area represents the relatively small impact on Δ C s,τ of differences in modelled spatial climate change patterns at 2 °C of global warming. In order to estimate the remaining uncertainty in Δ C s,τ , we treat this spread as equivalent to an observational uncertainty in an emergent constraint approach [26] . We apply a standard statistical approach [27] , [28] to estimate the probability density function of the y -axis variable (model Δ C s,τ ), accounting for both this observational spread and the quality of the emergent relationship. To test the robustness to the choice of observations we have repeated the analysis with different datasets that represent heterotrophic respiration, which produces strongly-overlapping emergent constraints, and completing the analysis with both CMIP6 and CMIP5 models shows that the result is also robust to the choice of model ensemble (see Table 1 ). Figure 4 b shows the resulting emergent constraint (blue line), and compares to the unweighted histogram of model values (grey blocks), and a Gaussian fit to that prior distribution (black line). The spatial emergent constraint reduces the uncertainty in Δ C s,τ at 2 °C of global warming from −196 ± 117 PgC to −232 ± 52 PgC (where these are mean values plus and minus one standard deviation for the top 1 metre). This same method can be applied to find constrained values of Δ C s,τ for other values of global warming. Figure 4 c shows the constrained range of Δ C s,τ as a function of global warming. This rules out the most extreme projections but nonetheless suggests substantial soil carbon losses due to climate change even in the absence of losses of deeper permafrost carbon. Obtaining spatial relationships In this section we explain how the quadratic relationships representing the spatial \(\mathrm{log}\,{\tau }_{{\rm{s}}}\) -temperature sensitivity shown in Fig. 3 a (and Supplementary Figs. 2 , 3 and 6 ) were derived, for both the Earth System Models (ESMs) in CMIP6 and CMIP5, and using the observational data. This is similar to the method used in Koven et al. [16] . Obtaining spatial relationships for CMIP models The CMIP6 models used in this study are shown in the Table 2 , and the CMIP5 models used in this study are shown in Table 3 . Table 2 CMIP6 models. Full size table Table 3 CMIP5 models. Full size table To obtain model specific spatial \(\mathrm{log}\,{\tau }_{{\rm{s}}}\) -temperature relationships, the following method was used. A reference time period was considered (1995–2005), this was taken as the end of the CMIP5 historical simulation to be consistent across CMIP generations and to best match the observational data time frame considered. Then, monthly model output data was time averaged over this period, for the output variables ‘soil carbon content’ ( C s ) in kg m −2 , ‘heterotrophic respiration carbon flux’ ( R h ) in kg m −2 s −1 , and ‘air temperature’ in K. The variables C s and R h were used to obtain values for soil carbon turnover time ( τ s ) in years, using the equation τ s = C s /( R h × 86400 × 365). The model temperature variable units were converted from K to °C. For each model, these values of \(\mathrm{log}\,{\tau }_{{\rm{s}}}\) were plotted against the corresponding spatial temperature data to obtain the spatial \(\mathrm{log}\,{\tau }_{{\rm{s}}}\) -temperature plot. Then, quadratic fits (using the python package numpy polyfit) are calculated for each model, which represent the spatial \(\mathrm{log}\,{\tau }_{{\rm{s}}}\) relationship and sensitivity to temperature. These model specific relationships are shown by the coloured lines in Fig. 3 a in the main manuscript, and in Supplementary Fig. 2 for CMIP6 and in Supplementary Fig. 3 for CMIP5. Obtaining spatial relationships for observations Following Koven et al. [16] , we estimated observational soil carbon data (to a depth of 1 m) by combining the Harmonized World Soils Database (HWSD) [19] and Northern Circumpolar Soil Carbon Database (NCSCD) [20] soil carbon datasets, where NCSCD was used where overlap occurs. To calculate soil carbon turnover time, τ s , using the following equation: τ s = C s / R h , we require a global observational dataset for heterotrophic respiration. In the main manuscript, CARDAMOM (2001–2010) heterotrophic respiration ( R h ) is used [21] . We completed a sensitivity study on the choice of observational heterotrophic respiration dataset, see below. The WFDEI dataset is used for our observational air temperatures (2001–2010) [24] . Then, these datasets can be used to obtain the observational \(\mathrm{log}\,{\tau }_{{\rm{s}}}\) -temperature relationship, using the same quadratic fitting as with the models. This represents the ‘real world’ spatial temperature sensitivity of \(\mathrm{log}\,{\tau }_{{\rm{s}}}\) , and is shown by the thick-dotted-black line in Fig. 3 a of the main manuscript. A comparison of the derived observational relationships can be seen in Supplementary Fig. 6 . Observational sensitivity study We completed a sensitivity study to investigate our constraint dependence on the choice of observational heterotrophic respiration dataset (CARDAMOM (2001–2010) [21] ). The other observational datasets considered are as follows: NDP-08 ‘Interannual Variability in Global Soil Respiration on a 0.5 Degree Grid Cell Basis’ dataset (1980–1994) [29] , ‘Global spatiotemporal distribution of soil respiration modelled using a global database’ [30] , and MODIS net primary productivity (NPP) (2000–2014) [31] . Supplementary Fig. 4 shows scatter plots showing one-to-one comparisons of these observational datasets against one another, and Supplementary Fig. 5 shows the corresponding comparisons of the equivalent \(\mathrm{log}\,{\tau }_{{\rm{s}}}\) values calculated from each dataset. The CARDAMOM R h dataset is used in the main manuscript for the following two main reasons: firstly, we calculate τ s using heterotrophic respiration which allows for consistency between models and observations, and secondly, the dataset does not use a prescribed q 10 sensitivity [21] . Instead, the CARDAMOM R h dataset was derived by explicitly assimilating observations into a process-based diagnostic land-surface model. To test the robustness of our results, we also repeated our analysis with MODIS NPP and Raich 2002, for both CMIP6 and CMIP5 together, and as separate model ensembles. Supplementary Fig. 6 shows the observational \(\mathrm{log}\,{\tau }_{{\rm{s}}}\) -temperature relationships, derived using each of these observational datasets. The results are presented in Table 1 which shows the constrained values of Δ C s,τ at 2 °C global mean warming. We decided not to complete the paper analysis using the Hashimoto dataset since not only is it inconsistent with the three other datasets considered, it also shows an arbitrary maximum respiration level (Supplementary Fig. 4 ), which likely results from the assumed temperature-dependence of soil respiration in this dataset which takes a quadratic form [30] . The quadratic form is justified based on a site-level study in which it is used to fit temporal dynamics. However, the parameters for the quadratic function that are fitted in the Hashimoto study are very different from those in the site-level study, which therefore suggests that the same relationship does not apply to the global distribution of mean annual soil respiration. Equation for the soil carbon turnover time component of soil carbon change The equation used in this study for the component of the change in soil carbon (Δ C s ) due to the change in soil carbon turnover time (Δ τ s ) was derived in the following way. Starting with the equation for soil carbon (based on the definition of τ s ): 
    C_s=R_h τ_s
 (2) As discussed in the main manuscript, we can write this change in soil carbon (Δ C s ), as the sum of a term arising from changes in litter-fall (Δ C s,L ), and a term arising from changes in the turnover time of soil carbon (Δ C s,τ ): 
    ΔC_s= Δ(R_h τ_s)≈ΔC_s,L(t)+ΔC_s,τ(t) = τ_s,0 ΔR_h(t)+R_h,0 Δτ_s(t)
 (3) Hence, the equation for the component of soil carbon change due to the change in τ s is: 
    ΔC_s,τ=R_h,0 Δτ_s
 (4) In this study we use R h from the reference period (‘present day’), which we call R h,0 , to allow us to investigate the response of Δ C s,τ as a result of the response of τ s to climate change. Modelled future temperature The proof of principle figure (Fig. 3 b) considers ΔC s,τ between the end of the 21st century (2090–2100), for each future SSP scenario (SSP126, SSP245, SSP585) [22] or equivalent future RCP scenario (RCP2.6, RCP4.5 and RCP8.5) [23] , and our reference period from the historical simulation (1995–2005), for each CMIP6 ESM and CMIP5 ESM, respectively. To consider specific °C of global warming (Fig. 4 ), the future spatial temperature profiles at these specific global mean warming levels, for example: 1 °C, 2 °C and 3 °C global mean warming, were calculated as follows. The temperature change is calculated from our reference period (1995–2005), and then a 5-year rolling mean of global mean temperature is taken to remove some of the interannual variability. Once the year that the given temperature increase has been reached is obtained, a time average including −5 and +5 years is taken, and the spatial temperature distribution of that model averaged over the deduced time period is used for the calculations of future τ s . Anomaly correction for future temperature projections To remove uncertainty due to errors in the models’ historical simulation, a spatial future temperature anomaly was projected using each model and each respective future SSP/RCP scenario separately. To calculate this, the temperature at the reference time frame (1995–2005), which overlaps the WFDEI observational temperature data time frame (2001–2010), is subtracted from the future temperature profile for each model (as calculated above), to calculate the temperature change. Then, this temperature anomaly is added onto the observational temperature dataset to give a model-derived future ‘observational’ temperature for each model. Proof of concept for our method Our method relies on the idea that the spatial temperature sensitivity can be used to project and constrain the temporal sensitivity of τ s to temperature, and subsequently global warming. To test the robustness of this method, Δ C s,τ calculated using model Δ τ s , and temperature sensitivity relationship-derived Δ τ s , are compared. The change in soil carbon turnover time (Δ τ s ) was either calculated using model output data to obtain model-derived Δ τ s as follows: 
    Δτ_s=τ_s^f-τ_s^h
 (5) where, 
    τ_s=C_s/R_h
 (6) Or calculated using the derived quadratic \(\mathrm{log}\,{\tau }_{{\rm{s}}}\) -temperature relationships to obtain relationship-derived Δ τ s , which is based on the following equation: 
    Δτ_s=exp (p(T^f))-exp (p(T^h))
 (7) where, T is near surface air temperature, and T f represents a future temperature, and T h represents historical (present day) temperature from our reference period (1995–2005). The exponentials ( \(\exp\) ) are taken to turn \(\mathrm{log}\,{\tau }_{{\rm{s}}}\) values to τ s values. p( T ) represents the quadratic \(\mathrm{log}\,{\tau }_{{\rm{s}}}\) -temperature relationship as a function of temperature to obtain our estimated \(\mathrm{log}\,{\tau }_{{\rm{s}}}\) . These Δ τ s values are then put back into the Eq. ( 4 ) (with model-specific R h,0 ) to obtain the corresponding Δ C s,τ values. The proof of principle figure (Fig. 3 b) investigates the robustness of our method, where projections of model and relationship-derived values of Δ C s,τ are compared, and an r 2 value of 0.90 is obtained. The correlation of the data was also tested when investigating different levels of global mean warming to obtain the constrained values (Fig. 4 ). The r 2 values for were as follows: 1 °C is 0.84, 2 °C is 0.87 and 3 °C is 0.87. Calculating constrained values To obtain the constrained values of Δ C s,τ , the model-derived future ‘observational’ temperature for each model is used together with the observational derived \(\mathrm{log}\,{\tau }_{{\rm{s}}}\) -temperature relationship, to project values for future τ s . Then this together with relationship-derived historical τ s deduced using the observational temperature dataset, can be used to calculate Δ τ s . Finally global Δ C s,τ can be obtained by multiplying Δ τ s by the observational dataset for R h,0 (using Eq. ( 4 )), and then calculating a weighted-global total. As each model-derived future ‘observational’ temperature is considered separately, we obtain a range of projected observational-constrained Δ C s,τ values. We have now obtained a set of x and y values, corresponding to the relationship-derived and modelled values of Δ C s,τ , respectively, for each ESM. Where we have an x and y value for each model, representing the modelled Δ C s,τ ( y values), and the model specific relationship-derived Δ C s,τ ( x values). We also have an x obs value representing the mean observational-constrained Δ C s,τ value, and a corresponding standard deviation due to the uncertainty in the modelled spatial profiles of future temperatures. We follow the method used in Cox et al. 2018, which can be seen in the ‘Least-squares linear regression’ section and the ‘Calculation of the PDF for ECS’ section of the methods from this study [32] . Using this method, we obtain an emergent relationship between our x and y data points, which we can use together with our x obs and corresponding standard deviation to produce a constraint on our y -axis. This is shown in Fig. 4 a. From this we obtain a constrained probability density function on Δ C s,τ , with a corresponding uncertainty bounds which we consider at the 68% confidence limits (±1 standard deviation). Figure 4 b show the probability density functions representing the distribution of the range of projections, before and after the constraint. This method allows us to calculate a constrained probability density function on Δ C s,τ at each °C of global mean warming, using the data seen in Fig. 4 a for 2 °C warming, and our corresponding constrained values for 1 °C and 3 °C warming. Figure 4 c shows the resultant constrained mean value of Δ C s,τ obtained for each °C of global mean warming, and the corresponding uncertainty bounds at the 68% confidence limits (±1 standard deviation). Calculating effective q 10 for change in soil carbon Simple models of soil carbon turnover are often based on just a q 10 function, which means that τ s depends on temperature as follows: 
    τ_s=τ_s,0exp((-0.1 log q_10)Δ T)
 (8) We compared the results for Δ C s,τ that would be derived from a simple q 10 function with our emergent constraint results for Δ C s,τ , to estimate an effective q 10 sensitivity of heterotrophic respiration. To do this, we can obtain an equation for Δ τ s derived from Eq. ( 8 ). This is done by considering the following, where τ s,0 is an initial τ s , we can substitute in τ s in temperature sensitivity form to obtain an equation for Δ τ s in temperature sensitivity form: 
    Δτ_s=τ_s-τ_s,0
 (9) 
    Δτ_s=τ_s,0exp((-0.1 log q_10)Δ T)-τ_s,0
 (10) Then, we can substitute this Δ τ s into Eq. ( 4 ) and simplify to obtain an equation relating Δ C s,τ and Δ T : 
    ΔC_s,τ=R_h,0τ_s,0[exp ((-0.1 log q_10)Δ T)-1]
 (11) 
    ΔC_s,τ=C_s,0[exp ((-0.1 log q_10)Δ T)-1]
 (12) This equation was used to calculate different Δ C s,τ –Δ T sensitivity curves based on different values on q 10 , for example q 10 = 2, with different amounts of global mean warming to represent Δ T , and initial observational soil carbon stocks C s,0 . These curves can be seen on Figs. 1 b and 4 c. Note that there is no direct relationship between the effective q 10 for soil carbon change shown in Figs. 1 b and 4 c, and the spatial τ s –T relationships in Fig. 3 a. Our q 10 value is an effective q 10 value that indicates the sensitivity of global soil carbon (in the top 1 metre) to global mean temperature.